Lonsdaleite is faulted and twinned cubic diamond and does not exist as a discrete material Lonsdaleite, also called hexagonal diamond, has been widely used as a marker of asteroidal impacts. It is thought to play a central role during the graphite-to-diamond transformation, and calculations suggest that it possesses mechanical properties superior to diamond. However, despite extensive efforts, lonsdaleite has never been produced or described as a separate, pure material. Here we show that defects in cubic diamond provide an explanation for the characteristic d -spacings and reflections reported for lonsdaleite. Ultrahigh-resolution electron microscope images demonstrate that samples displaying features attributed to lonsdaleite consist of cubic diamond dominated by extensive {113} twins and {111} stacking faults. These defects give rise to nanometre-scale structural complexity. Our findings question the existence of lonsdaleite and point to the need for re-evaluating the interpretations of many lonsdaleite-related fundamental and applied studies. The allotropes of carbon display a wide diversity of structures that include the three-dimensional (3D) diamond and graphite, two-dimensional (2D) graphene and curved nanotubes and fullerenes. Within this diversity are materials with extraordinary properties, paramount being cubic diamond, which has the highest known hardness and thermal conductivity. Diamond is reported to have a number of polytypes, of which lonsdaleite (also called hexagonal diamond) has received particularly intense attention. Lonsdaleite was first described almost 50 years ago from the Canyon Diablo iron meteorite [1] , [2] . Its formation was attributed to shock-induced transformation of graphite within the meteorite upon impact with Earth, and its occurrence was used as an indicator of shock [1] , [2] , [3] . It has since been reported from several meteorites as well as from terrestrial sediments and has been attributed to asteroidal impacts, both extraterrestrial and on Earth [4] , [5] , [6] , [7] . Lonsdaleite was proposed to have a wurtzite (ZnS)-type structure with space group P6 3 /mmc ( a =0.251 and c =0.412 nm) and with all structural positions occupied by carbon [1] , [2] , [3] , [8] . Observations and theoretical studies suggested a structural relationship among graphite, cubic diamond and lonsdaleite and an important role of the latter during the graphite-to-diamond transition [3] , [9] , [10] , [11] , [12] , [13] , [14] . Furthermore, an area centred around 18 GPa and 1,400 K in the pressure–temperature diagram for carbon was attributed to a phase called ‘retrievable hexagonal-type diamond’ [10] , which corresponds to the conditions where lonsdaleite has been reported [3] , [11] , [15] . Lonsdaleite has also received much attention because of its potentially superior mechanical properties, such as compressive strength, hardness and rigidity, thought to rival or exceed those of cubic diamond [16] , [17] . However, these exceptional properties have not been proven experimentally because of the inability to synthesize lonsdaleite as a pure phase. It has been reported to form during static compression of graphite [3] , [9] , [13] , [15] , [16] , [17] , [18] ; high-pressure–high-temperature treatment of powdered diamond, graphite and amorphous carbon [19] ; explosive detonation and shock compression of graphite [11] , [20] and diamond [21] ; and chemical vapour deposition of hydrocarbon gases [22] ; however, in all cases the synthesis product also contained cubic diamond, graphite or both. Published powder X-ray diffraction (XRD) patterns of lonsdaleite show peaks of cubic diamond plus extra, very broad and poorly resolved maxima at 0.218, 0.193, 0.151 and 0.116 nm that have been indexed using a hexagonal unit cell [1] , [2] , [3] , [14] , [15] , [20] . However, these maxima either occur on the shoulders of diamond peaks ( Fig. 1a,b ) or match those of graphite, but well-resolved X-ray reflections for lonsdaleite have not been reported. Selected-area electron diffraction (SAED), Raman, electron energy-loss spectroscopy (EELS) and high-resolution transmission electron microscopy have also been used for identification of lonsdaleite [4] , [5] , [6] , [7] , [14] , [15] , [18] , [23] , [24] ; however, interpretation of data is ambiguous ( Supplementary Note 1 ). In spite of the many diffraction and spectroscopic studies, unambiguous data that prove the existence of lonsdaleite as a distinct material have not been reported. 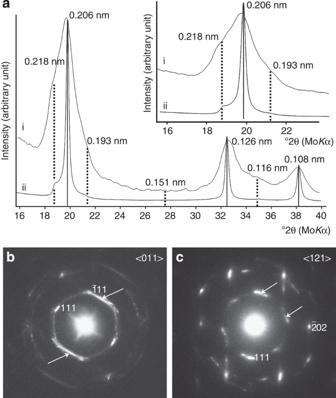Figure 1: XRD and SAED patterns from the Canyon Diablo and synthetic samples. They show features reported for ‘lonsdaleite’1,2,3,4,5,6,7,14,15,19,20. (a) XRD patterns from (i) Canyon Diablo and (ii) synthetic sample. Cubic diamond reflections are marked with solid black lines. The positions attributed to lonsdaleite are indicated by vertical dotted lines. (b) SAED pattern from Canyon Diablo sample, indexed as diamond along <011>. (c) SAED pattern from Canyon Diablo sample, indexed as diamond along <121>. The white arrows inbpoint to positions having ad-value of 0.218 nm (attributed to the 100 reflection of ‘lonsdaleite’), and those incmark hexagonally arranged reflections. SAED patterns with features matching those ofb,chave been interpreted as evidence for ‘lonsdaleite’ projected along <010> and <001>4,5,6,7,14,15,20, respectively. Figure 1: XRD and SAED patterns from the Canyon Diablo and synthetic samples. They show features reported for ‘lonsdaleite’ [1] , [2] , [3] , [4] , [5] , [6] , [7] , [14] , [15] , [19] , [20] . ( a ) XRD patterns from (i) Canyon Diablo and (ii) synthetic sample. Cubic diamond reflections are marked with solid black lines. The positions attributed to lonsdaleite are indicated by vertical dotted lines. ( b ) SAED pattern from Canyon Diablo sample, indexed as diamond along <011>. ( c ) SAED pattern from Canyon Diablo sample, indexed as diamond along <121>. The white arrows in b point to positions having a d -value of 0.218 nm (attributed to the 100 reflection of ‘lonsdaleite’), and those in c mark hexagonally arranged reflections. SAED patterns with features matching those of b , c have been interpreted as evidence for ‘lonsdaleite’ projected along <010> and <001> [4] , [5] , [6] , [7] , [14] , [15] , [20] , respectively. Full size image Here we provide a new explanation, based on faulted and twinned cubic diamond, for the diffraction features attributed to lonsdaleite. Because we question its existence, we will hereafter refer to it as ‘lonsdaleite’ to indicate scepticism that it exists as a discrete material. XRD and SAED patterns, EELS data and scanning transmission electron microscope (STEM) images of natural samples ( Supplementary Fig. 1 ) from the Canyon Diablo meteorite, the type specimen from which ‘lonsdaleite’ was first described [1] , [2] , and of synthetic material ( Supplementary Fig. 1 ) prepared under conditions where ‘retrievable hexagonal-type diamond’ was reported [10] , support our argument. The finding calls for re-evaluation of previous reports regarding ‘lonsdaleite.’ ‘Lonsdaleite’ diffraction features The XRD patterns of Canyon Diablo diamonds and the synthetic material display the poorly resolved diffraction maxima attributed [1] , [2] , [3] , [14] , [15] , [19] , [20] to ‘lonsdaleite’ ( Fig. 1a ). The SAED patterns of numerous grains consist of either spotty rings with streaking and smeared intensities or reflections arranged nearly hexagonally ( Figs 1b,c and 2a ). These patterns are consistent with diamond projected along <011> or <121>, respectively, although the streaking and hexagonally arranged 111 reflections are incompatible with defect-free single-crystal cubic diamond. Such data have been interpreted as evidence for ‘lonsdaleite’ projected along <010> and <001> [4] , [5] , [6] , [7] , [14] , [15] , [20] . The circularly integrated intensity profiles of these SAED patterns ( Supplementary Fig. 2 ) match the profile of the XRD pattern and show peaks for cubic diamond together with poorly resolved maxima at the d -spacings attributed to ‘lonsdaleite.’ In order to understand the structural features that give rise to these reflections and their d- spacings, we imaged these samples using a state-of-the-art ultrahigh-resolution STEM. 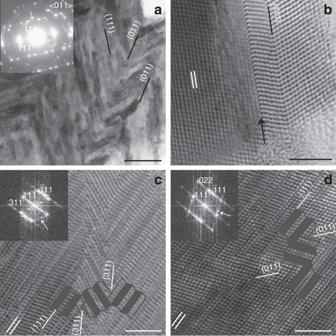Figure 2: STEM images provide evidence for stacking faults and multiple types of twins. These defects give rise to the diffraction features attributed to ‘lonsdaleite.’ (a) Low-magnification STEM image and corresponding SAED pattern (inset) from the synthetic sample. Black lines and symbols in the image indicate twin planes. Inamultiple {111} twins (indicated by black and white bands) give rise to {011} twins. The white arrow in the insert points to the position having ad-value of 0.218 nm that has been attributed to the 100 reflection of ‘lonsdaleite.’ (b) A (111) twin (black line) and a (111) stacking fault (indicated by a black arrow) in the synthetic sample. The 0.206-nm {111} fringes are marked with white parallel lines here and elsewhere. (c) {113} twins with corresponding FFT (insert) for the Canyon Diablo sample. (d) {011} twins with corresponding FFT (insert) for the Canyon Diablo sample. {111} stacking faults result in streaking of reflections in the SAED pattern and FFTs. Inc,d, multiple {111} twins (indicated by shaded overlays) give rise to the {113} and {011} twins. These twins result in the characteristic SAED ring patterns (Figs 1band2a) as they give rise to additional streaking, respectively, at 59° (white arrow on FFT inc) and 71° (white arrow on FFTs ind) to the strong {111} streaking. Scale bars mark 200 nm foraand 2 nm forb–d. Figure 2: STEM images provide evidence for stacking faults and multiple types of twins. These defects give rise to the diffraction features attributed to ‘lonsdaleite.’ ( a ) Low-magnification STEM image and corresponding SAED pattern (inset) from the synthetic sample. Black lines and symbols in the image indicate twin planes. In a multiple {111} twins (indicated by black and white bands) give rise to {011} twins. The white arrow in the insert points to the position having a d -value of 0.218 nm that has been attributed to the 100 reflection of ‘lonsdaleite.’ ( b ) A (111) twin (black line) and a (111) stacking fault (indicated by a black arrow) in the synthetic sample. The 0.206-nm {111} fringes are marked with white parallel lines here and elsewhere. ( c ) {113} twins with corresponding FFT (insert) for the Canyon Diablo sample. ( d ) {011} twins with corresponding FFT (insert) for the Canyon Diablo sample. {111} stacking faults result in streaking of reflections in the SAED pattern and FFTs. In c , d , multiple {111} twins (indicated by shaded overlays) give rise to the {113} and {011} twins. These twins result in the characteristic SAED ring patterns ( Figs 1b and 2a ) as they give rise to additional streaking, respectively, at 59° (white arrow on FFT in c ) and 71° (white arrow on FFTs in d ) to the strong {111} streaking. Scale bars mark 200 nm for a and 2 nm for b – d . Full size image The STEM images of the samples differ from well-ordered cubic diamond by displaying prominent chevron patterns and features that arise from multiple twins and stacking faults ( Figs 2 , 3 , 4 , Supplementary Fig. 3 ). The twins in the Canyon Diablo sample divide the grains into domains that are 1- to 3-nm wide ( Fig. 2 ), and the stacking faults produce domains two to four layers across (0.4–0.8 nm wide; Fig. 3 ). The synthetic sample shows a similar domain structure, although the domains are wider (2–20 nm), and there are fewer stacking faults. The C K-edge EELS data from the structurally complex areas are consistent with sp 3 -bonded carbon and are indistinguishable from cubic diamond ( Supplementary Fig. 4 ). 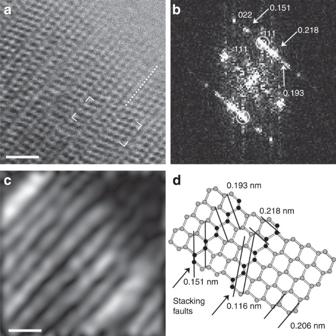Figure 3: Stacking faults provide an explanation for the reflections andd-spacings of ‘lonsdaleite.’ (a) <011> STEM image from the Canyon Diablo sample; one of many {111} stacking faults is indicated by the dotted white line. (b) FFT calculated froma. White arrows indicate spacings (0.218, 0.193 and 0.151 nm) that have been attributed to ‘lonsdaleite’. (c) Amplitude image calculated from the {−111} set of diamond reflections (white circles inb). Bright regions indicate domains two to four layers across separated by {111} stacking faults. (d) Structure model of the region marked with white corners ina. Stacking faults (black layers of atoms) result ind-spacings that are absent in single-crystal diamond and give rise to the broad X-ray and electron-diffraction features. Scale bars mark 1 nm fora,c. A question thus arises about how to explain the reflections and d- spacings of ‘lonsdaleite?’ Figure 3: Stacking faults provide an explanation for the reflections and d- spacings of ‘lonsdaleite.’ ( a ) <011> STEM image from the Canyon Diablo sample; one of many {111} stacking faults is indicated by the dotted white line. ( b ) FFT calculated from a . White arrows indicate spacings (0.218, 0.193 and 0.151 nm) that have been attributed to ‘lonsdaleite’. ( c ) Amplitude image calculated from the {−111} set of diamond reflections (white circles in b ). Bright regions indicate domains two to four layers across separated by {111} stacking faults. ( d ) Structure model of the region marked with white corners in a . Stacking faults (black layers of atoms) result in d -spacings that are absent in single-crystal diamond and give rise to the broad X-ray and electron-diffraction features. Scale bars mark 1 nm for a , c . 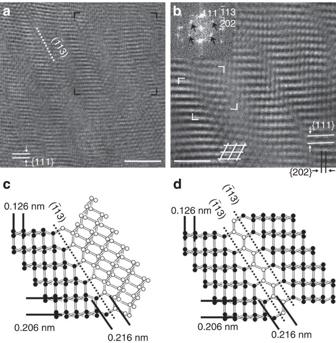Figure 4: Twins provide an alternate explanation for the diffraction features of ‘lonsdaleite.’ (a) <121> STEM image from the Canyon Diablo sample; one of many {113} twins is indicated by the dotted white line. (b) Background-filtered image calculated from the region marked by black corners ina. Intersecting white lines inbmark domains separated by regions that exhibit hexagonal fringes. The FFT in the insert shows hexagonally arranged reflections (black arrows) that are absent in single-crystal diamond. (c) Structure model of the {113} diamond twin. The structure across the twin consists of hexagonally arranged carbon atoms. Black and white atoms indicate twin domains. (d) Structure model of the region marked with white corners inb. The figure shows two layers of hexagonally arranged carbon atoms with 0.216-nm spacings, equivalent to two 0.108-nm {113} planes, which matches thed-value of 100 reflection attributed to ‘lonsdaleite.’ Scale bars mark 2 nm foraand 1 nm forb. Full size image Figure 4: Twins provide an alternate explanation for the diffraction features of ‘lonsdaleite.’ ( a ) <121> STEM image from the Canyon Diablo sample; one of many {113} twins is indicated by the dotted white line. ( b ) Background-filtered image calculated from the region marked by black corners in a . Intersecting white lines in b mark domains separated by regions that exhibit hexagonal fringes. The FFT in the insert shows hexagonally arranged reflections (black arrows) that are absent in single-crystal diamond. ( c ) Structure model of the {113} diamond twin. The structure across the twin consists of hexagonally arranged carbon atoms. Black and white atoms indicate twin domains. ( d ) Structure model of the region marked with white corners in b . The figure shows two layers of hexagonally arranged carbon atoms with 0.216-nm spacings, equivalent to two 0.108-nm {113} planes, which matches the d -value of 100 reflection attributed to ‘lonsdaleite.’ Scale bars mark 2 nm for a and 1 nm for b . Full size image Explanation of the ‘lonsdaleite’ diffraction features SAED patterns and STEM images along <011> and <121> of both the natural and synthetic samples demonstrate their structural complexity. The STEM images reveal two mechanisms that explain the features attributed to ‘lonsdaleite.’ Images along <011> show extensive {111} twinning (mechanism I), which results in abundant twin interfaces and stacking faults. These twins occur together with two new types of twins: {113} and {011} ( Figs 2 and 3 ). Although {113} diamond twins were proposed from molecular dynamics calculations [25] , they have not been reported experimentally. Observing the {113} twins requires resolving the 0.126-nm spacings, which was only possible with the ultrahigh resolution provided by an aberration-corrected microscope. The other new type of twin is {011} and it can be recognized from prominent chevron patterns in low-magnification images ( Fig. 2a ). We interpret the chevron twins as evidence for local regions lacking the symmetry of cubic diamond. The local symmetry loss is the result of multiple {111} twins and abundant stacking faults ( Fig. 2a,d ). The {111} stacking faults and twins interrupt the {111} periodicity ( Figs 2 and 3 ) and result in broad diffraction maxima at the d -spacings of ‘lonsdaleite’ on XRD ( Fig. 1a ) and SAED patterns ( Figs 1b and 2a ) as well as fast Fourier transforms (FFTs) ( Figs 2c,d and 3b ). The STEM images along <121> show evidence for another mechanism (mechanism II) that can explain the reported reflections and d -spacing of ‘lonsdaleite.’ The {113} twinning visible in the <121> projections results in prominent domains elongated parallel to {113} and recognized by their conspicuous {111} and perpendicular {022} fringes ( Fig. 4 , Supplementary Fig. 3 ). The domains are bordered by paired {113} twins. Adjacent {113} twins result in regions that are two-layer thick ( Fig. 4d ) and produce hexagonally arranged reflections in FFTs and SAED patterns ( Figs 1c and 4b , Supplementary Fig. 3 ). These twins result in a broad diffraction maximum at 0.216 nm, with hexagonally arranged carbon atoms across the twin boundary ( Fig. 4c,d , Supplementary Fig. 3c ). Consistent with prior work, discrete ‘lonsdaleite’ grains were not found; however, the above results provide a new interpretation of the observed diffraction features previously attributed to ‘lonsdaleite.’ We found its reported features on multiple XRD and SAED patterns; however, detailed STEM investigations showed no evidence for ‘lonsdaleite.’ The local arrangements of carbon atoms across the stacking faults and twin boundaries give rise to diffraction intensities with the d -spacings reported for ‘lonsdaleite’ ( Figs 3d and 4a , Supplementary Fig. 3 ). The subnanometre domains produce asymmetric broadening of diffraction peaks in XRD and SAED patterns. These observations are consistent with the proposed 111 diamond peak-broadening caused by stacking faults [26] , [27] , and are analogous to what occurs in face-centred cubic metals such as Co [28] . We provide new insights into the pressure–temperature phase diagram of carbon. The STEM images and diffraction patterns of the synthetic sample prepared through direct conversion from graphite and under conditions corresponding to ‘retrievable hexagonal-type diamond’ [10] show features consistent with cubic diamond twins and faults ( Fig. 2a,b , Supplementary Fig. 3 ). Therefore, we suggest that the region centred around 18 GPa and 1,400 K, actually corresponds to the field of cubic diamond containing defects in the form of twins and stacking faults. Furthermore, our results imply that graphite transforms to diamond without intermediate ‘lonsdaleite,’ which is consistent with the recent findings of shock-produced interstratified graphite and diamond [29] . The abundant stacking faults and twins in the impact-produced diamonds from the Canyon Diablo meteorite result from shock metamorphism of graphite [30] . Similar nanometre-scale structural complexity occurs in the synthetic sample, which was prepared through static compression. Since both samples contain the same structural features, the origin of the observed defect structure is not necessarily shock. In fact, extensive diamond twins have been reported from highly strained, mechanically twinned pink diamonds, which are thought to form as a result of plastic deformation in the mantle [31] . These features indicate that deformation may also produce diamond having high concentrations of planar defects. Theoretical predictions suggest outstanding mechanical properties for ‘lonsdaleite’ [16] , [17] . These predictions are based on the presumption of a periodic structure; however, a material with such periodicity has not been found. We demonstrate that the samples that show the characteristic diffraction features of ‘lonsdaleite’ display extensive diamond twins and stacking faults that divide the grains into subnanometre domains. Grain-size reduction is a powerful mechanism for improving the hardness of many materials, diamond among them [32] , [33] , [34] . Decreasing the domains’ size through defects may similarly contribute to strengthening of the materials. Thus, materials with the structural complexity similar to that of the studied Canyon Diablo meteorite samples can be candidates for synthetic products that possess exceptional mechanical properties for technological applications. Materials Diamond-bearing regions from the Canyon Diablo meteorite were reacted with dilute HCl for 2 days. The resulting insoluble material was washed several times with distilled water, dried and concentrated by centrifuging in a lithium heteropolytungstate solution (density 2.9 g ml −1 ) followed by washing in distilled water. As a result of these procedures, black adamantine grains with rhombohedral and cubic forms having size from 0.05 to 1 mm were obtained ( Supplementary Fig. 1 ). A 0.12 × 0.10 × 0.08-mm grain was mounted on a glass capillary and X-rayed with a Bruker SMART APEX single-crystal diffractometer employing Mo K α radiation, a graphite monochromator and a 2,000-K CCD detector (Arizona State University, USA). A data set was obtained by rotating the omega goniometer by one-degree per frame and by collecting intensities by scanning the frames for 1-min per/frame. The intensities of the data set were integrated and converted to a one-dimensional X-ray pattern. A synthetic sample was prepared in a 5,000-ton multi-anvil press ( Supplementary Fig. 1 ). The sample assembly consisted of a MgO (+5 weight% Cr 2 O 3 ) octahedron (18-mm edge length) containing a LaCrO 3 heater. A cylinder of high purity graphite was used as a starting material. The cylinder was enclosed in a Ta capsule, pressurized to 19 GPa and heated at 2,473 K for 5 min, the conditions that correspond to those reported by [7] , where ‘retrievable hexagonal-type diamond’ occurs. The temperature was monitored with a W 3 Re/W 25 Re thermocouple located axially with respect to the heater, with a junction close to the Ta capsule. Powder XRD from the synthetic sample was obtained using a high-brilliance Rigaku diffractometer (Mo K α radiation) equipped with Osmic focusing X-ray optics and Bruker Apex CCD detector (University of Bayreuth, Germany). The diffraction patterns were processed using the Fit2D software [35] . Transmission electron microscopy (TEM) and image processing Samples were crushed with a pestle and mortar. A droplet (ca. 2 μl) of the crushed grains in suspension in water was placed on a lacy-C-coated Cu TEM grid and dried. Bright-field STEM images, SAED patterns and EELS data were acquired from electron-transparent areas of the residue protruding into the holes of the lacy-C grid using an aberration-corrected JEOL ARM200F scanning TEM (Arizona State University, USA; 200 keV, 0.08-nm point resolution). FFTs obtained from the STEM images and background-filtered images were calculated using the Gatan Digital Micrograph 3.5 software. The amplitude image of Fig. 3c was generated from Fig. 3a following the method described in refs 36 , 37 , using routines written for the Digital Micrograph software and applying 0.06-nm −1 -size Lorentzian masks for the {−111} set of diamond reflections. The background-filtered image of Fig. 4b was obtained by applying 0.06-nm −1 -size Lorentzian masks for the hexagonally arranged reflections. How to cite this article : Németh, P. et al. Lonsdaleite is faulted and twinned cubic diamond and does not exist as a discrete material. Nat. Commun. 5:5447 doi: 10.1038/ncomms6447 (2014).